Rapid antibiotic susceptibility testing and species identification for mixed samples 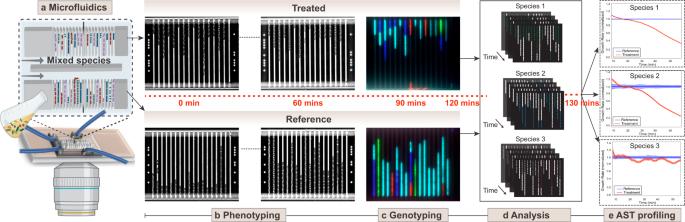Fig. 1: Schematic representation of the AST workflow with timeline. aA cartoon of the microfluidics setup with the mixed species loaded on the chip.bTime-lapse phase-contrast images of the cells in the traps when grown in media with (top) and without (bottom) antibiotics.cFluorescence images of the bacteria with ssDNA probes targeting the ribosomal RNA of specific bacteria for species identification.dAnalysis of time-lapse stacks and species ID using deep learning for segmenting and tracking cells.eDetection of AST profiles for individual pathogens at a given antibiotic concentration. Part of Fig. 1a created usingwww.biorender.com. Antimicrobial resistance is an increasing problem on a global scale. Rapid antibiotic susceptibility testing (AST) is urgently needed in the clinic to enable personalized prescriptions in high-resistance environments and to limit the use of broad-spectrum drugs. Current rapid phenotypic AST methods do not include species identification (ID), leaving time-consuming plating or culturing as the only available option when ID is needed to make the sensitivity call. Here we describe a method to perform phenotypic AST at the single-cell level in a microfluidic chip that allows subsequent genotyping by in situ FISH. By stratifying the phenotypic AST response on the species of individual cells, it is possible to determine the susceptibility profile for each species in a mixed sample in 2 h. In this proof-of-principle study, we demonstrate the operation with four antibiotics and mixed samples with combinations of seven species. The rapid increase in antibiotic resistance is a serious threat to human health; access to effective antibiotics is a cornerstone of modern medicine and a prerequisite for e.g. cancer treatment and surgery. Different investigations [1] , [2] make different estimations of how grave the situation is but there is a consensus view that action needs to be taken or the costs both in terms of human suffering and global economic impact will be staggering [3] . Experts also agree that the problem is at least partly due to indiscriminate use and misuse of a wide range of antibiotics [4] . To overcome this problem, personalized and rapid antibiotic susceptibility tests (ASTs) are needed, ideally at the point of care [5] . Without these tools, physicians are left with no other option than to prescribe broad-spectrum antibiotics in many cases since it can take several days to identify the pathogen(s) and the resistance profile. The limitations of conventional phenotypic ASTs (disk diffusion agar dilution or broth microdilution) are that they require bacterial growth for extended periods in the presence and absence of antibiotics to see an effect. However, for certain types of bacterial infections, even a delay of 6 h before treatment is initiated can have severe consequences [6] . One such example is sepsis, where the risk of death has been estimated to increase by 7.6% for every hour that effective treatment is not given [7] . Further, it is shown that in the absence of fast AST, more than 25% of septic patients were treated by clinicians with inappropriate antibiotics, which is strongly associated with mortality [8] , [9] , [10] . Thus, rapid and accurate ASTs are needed to save lives. But considering the increases in AMR, life-threatening conditions are not the main culprit, but rather the bulk usage of antibiotics for more benign conditions [11] . The exhaustion of effective antibiotics is also driven by the strategy to change first-line antibiotics when the local resistance prevalence has reached approximately 10–20%. If fast, reliable ASTs were accessible, high-resistance antibiotics could be used for 80–90% of the infections that are still susceptible. The obvious need and benefits of rapid AST, both for saving lives and guiding prescriptions, have resulted in the development of several new methods over the last decade. These methods are described in several recent reviews, e.g., [4] , [12] , and we will not repeat all the pros and cons of the different methods here. Briefly, these methods can be divided into two categories, genotypic and phenotypic. Genotypic methods identify specific genetic markers that are associated with antibiotic resistance. Although these methods can rapidly detect the presence of specific resistance genes, they depend on our knowledge of the resistance mechanisms which is far from complete [13] , in particular considering the rapid emergence of new resistance mechanisms. Furthermore, the absence of resistance genes does not predict susceptibility to antibiotics [14] , i.e., you may learn what not to use but not what will work. In phenotypic methods, the bacteria are exposed to an antibiotic and their phenotypic response, e.g., lysis or growth rate reduction, is monitored. Phenotypic methods work irrespective of the mechanism of resistance. If the phenotypic response is there, the bacterium is susceptible. The various rapid phenotypic ASTs that have reached the market can deliver an answer (susceptible or resistant) in 2–6 h for positive blood cultures that have been growing >6 h from sampling the patient. For other samples, e.g., urine, the time-to-answer can be reduced to 30 min for gram-negative species by loading the sample directly into a microchip and measuring the growth rate with and without antibiotics [15] . A limitation of all rapid phenotypic AST methods is that they only work if the species of the bacteria are known. Detailed species ID is not needed for infections with a narrow spectrum of pathogens [16] , but for sepsis and other more complex infections, it is essential. MALDI-TOF mass spec is currently the golden standard for species determination [17] . MALDI-TOF does however still require pre-culture of single bacterial species and may not work well for mixed infections commonly seen in sepsis, wounds, catheter-associated UTIs [18] , and community-acquired pneumonia, among others [19] . The challenge remains to make rapid phenotypic AST with species ID. To address this issue, we use a microfluidic chip to rapidly capture individual bacteria from a sample and optically monitor their growth with and without antibiotics. Next, we identify the bacterial species by fluorescence in situ hybridization (FISH) with species-specific ssDNA probes targeting the 16s/23s rRNA sequence. Once we have the species ID and AST response for each bacterium in the microfluidic chip, we stratify the AST response based on species, which implies that we can have samples with mixed species. A schematic overview of the approach is presented in Fig. 1 . Fig. 1: Schematic representation of the AST workflow with timeline. a A cartoon of the microfluidics setup with the mixed species loaded on the chip. b Time-lapse phase-contrast images of the cells in the traps when grown in media with (top) and without (bottom) antibiotics. c Fluorescence images of the bacteria with ssDNA probes targeting the ribosomal RNA of specific bacteria for species identification. d Analysis of time-lapse stacks and species ID using deep learning for segmenting and tracking cells. e Detection of AST profiles for individual pathogens at a given antibiotic concentration. Part of Fig. 1a created using www.biorender.com . Full size image In this proof of principle application, we perform the ASTs for seven common pathogens ( Escherichia coli , Klebsiella pneumonia, Pseudomonas aeruginosa, Proteus mirabilis , and Acinetobacter baumannii , as examples of gram-negative strains, and Enterococcus faecalis and Staphylococcus aureus as examples of gram-positives). We test four different antibiotics from different classes: Vancomycin (Van) [Glycopeptide], Ciprofloxacin (CIP) [Fluoroquinolones], Gentamicin (Gen) [an aminoglycoside], and Nitrofurantoin (NIT) [other agents]. Finally, we show how single-round, multi-color labeling enables the identification of up to ten species simultaneously. Phenotypic AST followed by Genotyping by FISH The culture chip that we have developed for this assay is capable of rapid capture of bacteria directly from a liquid sample and allows for optical monitoring of bacterial growth with and without antibiotics in real time. The same chip design has previously been used to capture bacteria from blood cultures despite an overwhelming excess of blood cells [20] . The chip features two rows of 3000 cell traps each. Each trap measures 1.25 × 1.25 × 50 μm [15] and has a constriction at the end which prevents the bacteria from escaping the trap while still allowing media and probes to flow around the cells. To simulate a mixed infection situation, bacterial overnight cultures of several different species were diluted in a Mueller Hinton (MH) broth, pooled, and directly loaded into the microfluidic chip. In a typical experiment, loading one or a few cells in each trap takes 1 min at ~10 5 CFU/ml. We supplied growth media with antibiotics to the traps in one of the two rows and plain growth media in the other. The phenotypic response to the antibiotic was determined in ≈60 min by capturing 100X phase-contrast images of each cell every 2 min and calculating the growth rates of individual cells in 10 min sliding windows. The phenotypic response can be pushed to shorter times depending on which antibiotics are used and at which concentration [15] . To identify the species of each bacterial cell, we performed fluorescence in situ hybridization (FISH) using species-specific, fluorescent ssDNA probes. These probes (Supplementary Data 1 ) bind to the abundant 16s/23s ribosomal RNA sequences and have previously been successfully used for species identification in positive blood cultures [21] . The species classification method for FISH signals is described in SI method 3 . Analysis using Deep learning models Performing growth-rates analysis on multi-species samples requires a general method for detecting and tracking cells that come in different shapes and sizes. In Delta 2.0 [22] , a U-net [23] was used to predict cell-vs-background maps of phase-contrast images and showed excellent performance for E. coli cells, both in mother-machine-like devices and on agarose pads. More general algorithms for cell segmentation, such as Cellpose [24] and its successor Omnipose [25] construct cell identities from intermediate fields (Fig. 2a ) learned by a convolutional neural network, similar to a U-net. Omnipose was shown to perform segmentation of bacterial cells independently of their morphology. Approaches that calculate cell identities (Cellpose, Omnipose) assign different unique labels to cells that share a boundary while cell-vs-background approaches (U-net) can not be used to separate cells that share a boundary. The former approaches require cell labels as training data while the latter needs only binary masks. Fig. 2: Analysis. a Omnipose network showing network structure, inputs, and outputs to the neural network and reconstruction of output to generate cell masks. b Quantified performance of cell segmentation in mother-machine devices. Average precision vs IOU threshold plot for mixed-species dataset. The IOU threshold defines valid matching between predicted mask and ground-truth masks, 0.5 indicating half the pixels were correctly matched and 1 indicating pixel perfect match for every cell. Average precision (TP / (TP + FP + FN)) is calculated from the valid matches (TP), no valid matches (FP), and the ground-truth masks that have no valid match (FN). c Few examples of phase-contrast images, ground-truths and network predictions of U-net and Omnipose. d Overview of tracker network. e Confusion matrix of the edge predictions. f Tracks of cells in one channel of the mother-machine device. Full size image A ground-truth training dataset (82 images) of mixed cells growing in mother-machine devices was created with human supervision using the LabelsToROIs tool [26] and custom scripts (SI method 1 ). We use an Omnipose model trained on this data for cell segmentation. Training and performance of Omnipose and U-net are also described in SI method 3 . The run-time performance of reconstruction steps from Omnipose network outputs was improved two-fold (SI Fig. 1b). Omnipose showed superior performance (Fig. 2b ) on mixed-species data compared to a U-net trained to predict binary masks. We showed that the omnipose performed equally well on mixed-species data as on data from pure E. coli cultures (SI Fig. 1b, e ); the performance of U-net, on the other hand, depended on the species. 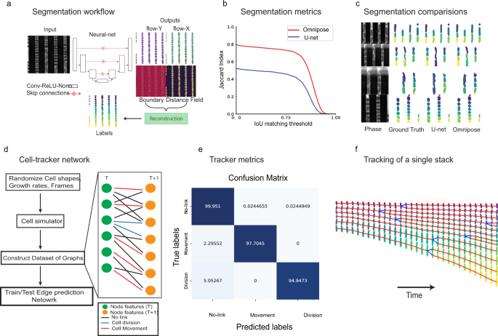Fig. 2: Analysis. aOmnipose network showing network structure, inputs, and outputs to the neural network and reconstruction of output to generate cell masks.bQuantified performance of cell segmentation in mother-machine devices. Average precision vs IOU threshold plot for mixed-species dataset. The IOU threshold defines valid matching between predicted mask and ground-truth masks, 0.5 indicating half the pixels were correctly matched and 1 indicating pixel perfect match for every cell. Average precision (TP / (TP + FP + FN)) is calculated from the valid matches (TP), no valid matches (FP), and the ground-truth masks that have no valid match (FN).cFew examples of phase-contrast images, ground-truths and network predictions of U-net and Omnipose.dOverview of tracker network.eConfusion matrix of the edge predictions.fTracks of cells in one channel of the mother-machine device. Figure 2c shows phase contrast images, their corresponding ground truths, and cells detected using Omnipose and U-net approaches, respectively. Previous approaches to successful E. coli tracking have constructed cell lineages using scoring mechanisms based on overlapping regions [27] or mother-daughter binary-mask predictions using the full features from the images [22] . The former approach is very sensitive to tuning overlap parameters while the latter is computationally expensive when a lot of small cells are present in the data. Inspired by recent developments in using Siamese networks [28] and graph formulations [29] for general object-tracking, we have now developed an approach that performs cell tracking using a network that compares cell properties between two frames and predicts the presence and type of connections, e.g., cell growth or division event (Fig. 2d ). Training data for this network was obtained using a simulator (SI method 4 ) that simulates cells of various kinds and growth rates growing in mother-machine channels. The training of the tracking network is described in the Supplementary information ( SI method 4) . In Fig. 2e , we show the confusion matrix of the model used for tracking experimental data evaluated on 100 randomly generated time-series stacks. Before constructing the tracks, the links that have abrupt increases in areas were removed as they correspond to merge events caused by segmentation errors (SI method 4 ). Figure 2f (left) shows a single segmented mother-machine trap tracked through time with growth/movement links (red) and division links (blue). Species assignment to tracks based on the species ID identified in the last frame was performed after cell-tracking (SI method 5 ). Species-wise AST response With the species ID and AST response for each cell in the microfluidic chip, the species-specific AST response could be determined in the mixed samples. Here, we first demonstrate the capability of the method to characterize a mixed sample of four different species, although clinical patient samples are more likely to contain only one or two [30] , [31] , [32] . The AST responses are shown in Fig. 3a–d . In each experiment, we obtained growth-response curves for three gram-negative strains ( Escherichia coli , Klebsiella pneumoniae , and Pseudomonas aeruginosa) and one gram-positive strain ( Enterococcus faecalis) . The experiments were performed with four different antibiotics: Vancomycin (Van) [Glycopeptide], Ciprofloxacin (CIP) [Fluoroquinolones], Gentamicin (Gen) [an aminoglycoside], and Nitrofurantoin (NIT) [other agents]. We present the results as response plots from individual experiments to simulate the clinical-sample situation. For comparison, we also display the average responses that would have been the result of the growth-rate measurements without species information. Successful AST profiling was achieved with samples containing as few as 100 bacteria/species. We used bacteria without specific resistance genes, but since some species have a natural resistance to specific antibiotics, the AST response varied with the species. 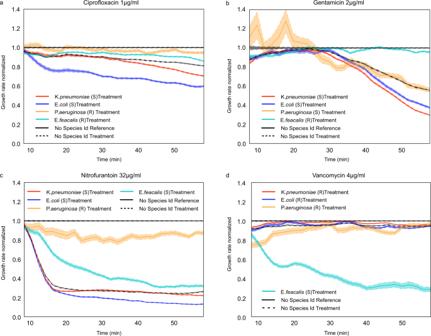Fig. 3: Species stratified responses to antibiotic treatments. a–dAST profiles with normalized growth rates for the four antibiotics used. The species stratified responses (mean and SEM), as well as the pooled response (without species stratification), are shown for each antibiotic. In all AST profile plots, S and R represent the Susceptible and Resistance, respectively. The experiment is performed once per antibiotic, although several non-reported experiments were performed for calibration. For example, Pseudomonas species are naturally resistant to Ciprofloxacin (Fig. 3a ) and Nitrofurantoin (Fig. 3b ), and their growth remained unaffected in the presence of 1 μg/ml Ciprofloxacin or 32 μg/ml Nitrofurantoin. The growth rate of the other bacterial species dropped more than 10% in 30 min in the presence of these drugs. Importantly, we see from the average, non-species-stratified data that without access to species ID, we would not have been able to detect the resistant Pseudomonas in the mixed population. Similarly, as expected, all species but E. faecalis were found to be susceptible to Gentamicin (2 μg/ml) (Fig. 3c ) and resistant to Vancomycin (4 μg/ml) (Fig. 3d ). Fig. 3: Species stratified responses to antibiotic treatments. a – d AST profiles with normalized growth rates for the four antibiotics used. The species stratified responses (mean and SEM), as well as the pooled response (without species stratification), are shown for each antibiotic. In all AST profile plots, S and R represent the Susceptible and Resistance, respectively. The experiment is performed once per antibiotic, although several non-reported experiments were performed for calibration. Full size image Scaling up FISH probing to 10 species It is estimated that >90% of clinical sepsis samples feature a subset of the 10 most frequent bacterial pathogens [33] . To increase the number of species that we can identify, we performed combinatorial FISH using a species-specific adaptor that can bind two different fluorescent oligo probes. With probes of four different colors, this set-up can identify up to 10 species (Fig. 4a ). We demonstrated the combinatorial FISH approach by identifying seven species loaded in the culture chip (Fig. 4b ). Species-wise combination of signals using all the adapters and probes are shown in SI Fig. 7 . Species classification was done using a random-forest classifier on the 4-d signal obtained from stacking images of four fluorescence channels (SI method 6 ). To demonstrate species-wise AST profiles using combinatorial FISH, we performed experiments with combinations of two species treated with different antibiotics (Fig. 5 ). For example, when Escherichia coli and Enterococcus faecalis were treated with Vancomycin (4 μg/ml), the two species showed clear, distinguishable growth-rate profiles corresponding to resistance and susceptibility, respectively (Fig. 5d ). Repeats for these experiments are shown in Fig. 5e–h . Fig. 4: Combinatorial FISH. a Overview of the combinatorial FISH probing for the multi species identification. A cartoon illustrating the different bacterial species with their ribosomal RNA (left). Illustration of the specific sequences with the multiple adapters targeting the ribosomal RNA of individual bacteria and its hybridization to the target rRNA (middle). Detection probes with different fluorophores. Hybridization of detection probes to the adapter sequences along with unique sequences that are targeted to the species specific rRNA (Right). b Example images (Scale bar 20 µm) of mixed species loaded in the microfluidic chip and probed using combinatorial FISH for species identification. After the hybridization step, cells were imaged in different channels (PhC, Alexa 488, Cy3, Cy5, and Texas Red). The bacterial species are marked in white ( Escherichia coli ), magenta ( Klebsiella pneumoniae ), cyan ( Pseudomonas aeruginosa ), brown ( Enterococcus faecalis ), yellow ( Acinetobacter baumannii ), navy blue ( Proteus mirabilis ) and red ( Staphylococcus aureus ). The experiment with all seven species mixed was performed a single time. However, similar experiments with all adaptors and probes mixed are reported in Fig. 5 . Full size image Fig. 5: Species-wise AST profiles for experiments with 2 species using the combinatorial FISH method. a P. aeruginosa and A. baumannii were treated with Gentamicin, b K. pneumoniae , and S. aureus treated with Ciprofloxacin, c E. coli , and P. mirabilis treated with Nitrofurantoin, d E. coli and E. faecalis treated with Vancomycin. e – h Biological repeats of 5a-5d, respectively. In all AST profile plots, S and R represent Susceptible and Resistance, respectively. Normalized growth rates ± SEM as a function of time are shown for each species detected in the experiments. Full size image In conclusion, we have demonstrated that it is possible to make rapid AST for mixed-species samples by performing sequential single-cell phenotypic susceptibility testing and fluorescence in situ hybridization in a microfluidic chip. Importantly, ID determination is also useful for non-mixed samples when it is essential to know which MIC breakpoints to use for making the SIR (susceptible-intermediate-resistant) call. Although species determination for non-mixed samples is possible by MALDI-TOF, it requires many more bacterial cells than direct single-cell imaging. Since antibiotic susceptibility breakpoints of closely related species are often the same, it can sometimes be enough to distinguish the bacterial family or genera. For example, an Enterobacteriales-specific color ID-code to cover Escherichia, Klebsiella , and Salmonella , which have very similar resistance breakpoints [34] . Different species-specific probes would in this case map the same color ID code, such that the ten codes can be used more efficiently. Similarly, we expect that it would be possible to have a common ID code for contaminant species, such that they are not mistaken for pathogens. However, if more than 10 specific ID codes are required, stripping and reprobing allow an exponential increase in how many classes can be identified [35] , [36] , but at the expense of time. In the current implementation, we ran the test one concentration at a time on a high-end research microscope and post-processed the imaging data. To make the technology useful in a clinical setting, data should be analyzed during the experiment and the fluidic chip should be parallelized to run multiple antibiotic concentrations simultaneously. Although we have not tested this type of setup in the present study, it should allow a MIC determination to identify intermediate isolates. A system with five different antibiotics at five different concentrations and a high level of automation has been developed for uncomplicated urinary tract infections [20] , which shows that upscaling to multiple testing conditions is possible. Finally, we would like to emphasize that the present study is proof of principle of combined phenotypic AST and species identification at the single-cell level. For this method to be clinically relevant, it needs to be calibrated and tested on many more clinical isolates as well as on real patient samples. Bacterial strains and antibiotics In this study, as a gram-negative representative we used E . coli K12 MG1655 (DA4201), K . pneumoniae (ATCC 13883), A. baumanni (DA68153), P. mirabilis (ATCC 29906) and P . aeruginosa (DA6215). As a gram-positive representative, we used E . faecalis (ATCC 51299) and S. aureus (ATCC 29213). We also used the fluorescently tagged P. aeruginosa (PAO1-GFP) cells, a kind gift from Oana Ciofu [37] . Antibiotics (Ciprofloxacin, Gentamicin, Nitrofurantoin, and Vancomycin) were purchased from Sigma-Aldrich. Stock solutions were prepared as per the supplier guidelines and stored at −20 °C. The solutions were thawed to room temperature before performing the AST experiments. We used concentrations of the antibiotics corresponding to the MIC values for E. coli (ATCC 25922) as defined by the European Committee on Antimicrobial Susceptibility Testing (EUCAST). We note that another, higher, concentration may be optimal to make a rapid SIR call. Media and culture conditions In all experiments, Mueller-Hinton (MH) medium (70192; Sigma-Aldrich) was used as a broth. Overnight cultures (ONC) were prepared by inoculating bacteria from glycerol stocks (−80 °C) in MH medium and incubating at 37 °C for 14–15 h with continuous shaking (200 rpm). From ONC, cells were diluted 1:1000 times into fresh MH medium supplemented with a surfactant (Pluronic F-108; 542342; Sigma-Aldrich; 0.085% (wt/vol) final concentration). The liquid culture was grown by shaking at 200 rpm at 37 °C for 2 h. Next, to perform AST experiments, we mixed the different strains in equal concentrations and loaded them on the microfluidic chip. The microfluidic chip and setup The chip consist of mainly two parts: a micromolded silicone elastomer [Sylgard 184; polydimethylsiloxane (PDMS)] and a 1.5 glass coverslip (Menzel-Gläser) which are covalently bonded together. Chip design and preparation were previously described in [15] , [38] . These references also describe the numbering of the ports used below. After punching the ports on the chip, it was placed on the microscope, and tubing (TYGON) was connected with a metal tubing connector. Briefly, cells were loaded using port 8.0 and port 2.0 was used for the exchange of medium with the probes. Ports 5.1, 5.2, and 6.0 were used for maintenance of back-channel pressure, and ports 2.1 and 2.2 were used for the supply of MH medium with and without the antibiotics at a pressure of 200 mbar. The pressure was controlled by an OB1-Mk3 regulator (Elveflow). Microfluidic experiments Imaging starts within five minutes after the supply of medium with and without the antibiotics to the cells. We used a Nikon Ti2-E inverted microscope equipped with a Plan Apo Lambda 100× oil immersion objective (Nikon). Images were captured by the Imaging Source (DMK 38UX304) camera. For phase contrast and fluorescence images, we used the optical setup as previously described in [15] , [38] and controlled by Micro-Manager [39] , and an in-house built plugin. We maintained 30 °C using a temperature controllable unit and a lexan enclosure (Oklab). Fast phenotypic AST The cells were loaded on the chip and exposed to growth media with and without the antibiotics in two different rows. In each row, a total of 70–80 positions, each including 16–21 cell traps, were images in the phase contrast channel (30 ms exposure time) every two minutes for an hour. Genotyping After phenotyping, the medium from ports 2.1 and 2.2 were depressurized to zero. To fix the cells, formaldehyde (4%) was added by switching the medium and applying pressure 200 mbar from port 2.0 for 4 min and subsequently washing the cells with 1 × phosphate-buffered saline (PBS) for 3 min. Cells were permeabilized by 70% EtOH for 4 min and washed with 1 × PBS (3 min). Cells were next treated with lysozyme (2 mg/ml) and lysostaphin (0.1 mg/ml) for 3 min and followed by quick washing with 1 × PBS for another 3 min. (Lysostaphin is only needed for S. aureus and was not used in Fig. 3 ). For species identification, we pooled all specific ssDNA probes (0.1 μM) (Supplementary Data 1 ) in a hybridization solution (30% formamide and 2 × SSC) and hybridized them for 30 min at 30 °C. In the case of the combinatorial method, we pooled all the detection probes (0.1 μM) (Supplementary Data 2 ) and species-specific adaptor sequences (Supplementary Data 3 ) in a hybridization solution (30% formamide and 2 × SSC) and hybridized them for 60 min at 30 °C. Next, we captured the fluorescence images for each probe in different channels (TYE 665, TYE 563, Texas Red, and Alexa Fluor 488) at 300 ms exposure times and respective phase contrast images at 30 ms exposure time. In total, it took 10–15 min to image all the positions in all the channels on the chip. Cell segmentation and channel detection Phase-Contrast images of the cells growing in channels were segmented for both cells and channels using a deep learning model with Omnipose method. 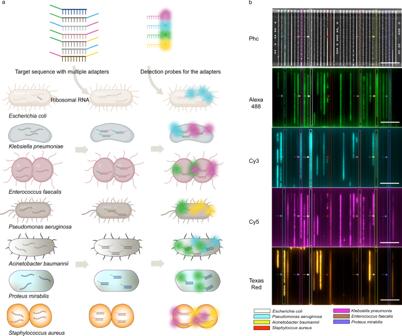Fig. 4: Combinatorial FISH. aOverview of the combinatorial FISH probing for the multi species identification. A cartoon illustrating the different bacterial species with their ribosomal RNA (left). Illustration of the specific sequences with the multiple adapters targeting the ribosomal RNA of individual bacteria and its hybridization to the target rRNA (middle). Detection probes with different fluorophores. Hybridization of detection probes to the adapter sequences along with unique sequences that are targeted to the species specific rRNA (Right).bExample images (Scale bar 20 µm) of mixed species loaded in the microfluidic chip and probed using combinatorial FISH for species identification. After the hybridization step, cells were imaged in different channels (PhC, Alexa 488, Cy3, Cy5, and Texas Red). The bacterial species are marked in white (Escherichia coli), magenta (Klebsiella pneumoniae), cyan (Pseudomonas aeruginosa), brown (Enterococcus faecalis), yellow (Acinetobacter baumannii), navy blue (Proteus mirabilis) and red (Staphylococcus aureus). The experiment with all seven species mixed was performed a single time. However, similar experiments with all adaptors and probes mixed are reported in Fig.5. 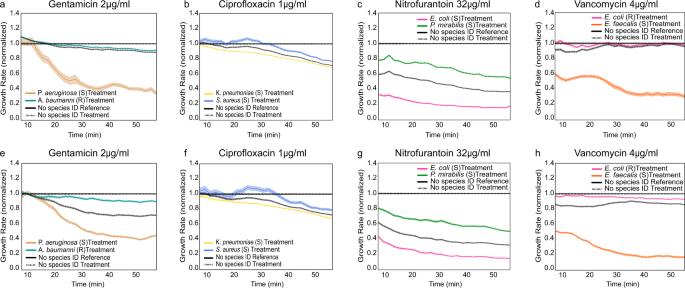Fig. 5: Species-wise AST profiles for experiments with 2 species using the combinatorial FISH method. aP. aeruginosaandA. baumanniiwere treated with Gentamicin,bK. pneumoniae, andS. aureustreated with Ciprofloxacin,cE. coli, andP. mirabilistreated with Nitrofurantoin,dE. coliandE. faecalistreated with Vancomycin.e–hBiological repeats of 5a-5d, respectively. In all AST profile plots, S and R represent Susceptible and Resistance, respectively. Normalized growth rates ± SEM as a function of time are shown for each species detected in the experiments. The cell-segmentation model was trained with data obtained from manually-labeled images of mixed species data and data obtained from E. coli (K12 MG1655 intC::P70-venusFast) that constitutively expresses mVenus. The training procedure was enhanced with data augmentations to force learning outputs of Omnipose network in different orientations and scales. The model training and performance compared to U-net is described in SI method 1 . The segmentation network performance on different species is also shown in SI method 1 . The channel segmentation model was trained with data that was refined based on histogram profiles, also described in SI method 2 . After obtaining channel locations, time-series stacks of segmented cells and corresponding fluorescent channel images were bundled for tracking, species assignment, and growth rate calculations. Cell tracking Cells were tracked through time using a neural network that scores links between cells from one frame to the next and predicts the type of link between them. Training data for cell tracking was obtained by simulating the growth of cells in mother-machine channels and is described in SI method 4 . Cells of different shapes, sizes, and growth rates were used to generate ground truths for the tracking network. Tracker network training and its performance are described in SI method 4 . The predictions of the network are cleaned for error using IoU (Intersection-over-Union) metric to remove spurious predictions. At test time, cells between frames were linked based on the probability scores, and tracks were generated by chaining a series of links. Cell tracks were corrected for errors (SI method 4 ). Species assignment and growth curve splitting For experiments where a single probe binds to a single species, fluorescent images for each mother machine channel were corrected for background, and continuous regions of signal above thresholds were mapped to species labels (SI method 3 ). Experiments with multiple fluorescent probes for a single species were classified using a Random-Forest classifier, described in SI method 6 . Continuous regions corresponding to one species (>90 pixels) were identified and bounding boxes were drawn around these regions. Cell tracks falling in these regions in the last frame before fixing cells were labeled with the corresponding species and all the species labels were rolled back to time point 0. Growth rates were calculated by fitting exponential curves on the areas of cells in a moving 5 timepoint window (SI method 7 ). Oligos and probes design FISH probe sequences for the individual target rRNA were obtained from the probeBase [21] , [40] , [41] and purchased from Integrated DNA Technologies ( www.idt.com ), see Supplementary data 1 . For the combinatorial FISH probing, we used barcode sequence and detection probes, which are listed in Supplementary Data 2 – 4 , purchased from IDT. Statistics and reproducibility All experiments were conducted using the same set-up. Both treated and reference cells used the same segmentation and tracking models. The experiments were not randomized. For growth rate measurements, each species’ growth rate was calculated using at least 100 cells. Cells with segmentation errors were not included in the growth-rate calculations. All AST profiles show normalized growth rates ± SEM. Detailed information on experimental repeats can be found in the individual figure legend. Reporting summary Further information on research design is available in the Nature Research Reporting Summary linked to this article.